IL-10 engages macrophages to shift Th17 cytokine dependency and pathogenicity during T-cell-mediated colitis Polymorphisms attenuating IL-10 signalling confer genetic risk for inflammatory bowel disease. Yet, how IL-10 prevents mucosal autoinflammation is incompletely understood. We demonstrate using lineage-specific deletions of IL-10Rα that IL-10 acts primarily through macrophages to limit colitis. Colitis depends on IL-6 to support pathologic Th17 cell generation in wild-type mice. However, specific ablation of macrophage IL-10Rα provokes excessive IL-1β production that overrides Th17 IL-6 dependency, amplifying the colonic Th17 response and disease severity. IL-10 not only inhibits pro-IL-1β production transcriptionally in macrophages, but suppresses caspase-1 activation and caspase-1-dependent maturation of pro-IL-1β to IL-1β. Therefore, lineage-specific effects of IL-10 skew the cytokine dependency of Th17 cell development required for colitis pathogenesis. Coordinated interventions may be needed to fully suppress Th17-mediated immunopathology. Inflammatory bowel diseases (IBDs), including Crohn’s disease and ulcerative colitis (UC), are characterized by chronic relapsing intestinal inflammation and disorganized immune responses in the gastrointestinal tract [1] . Although IBD pathogenesis is incompletely understood, mucosal T-helper type 17 (Th17) cells play a key pathologic role [2] , [3] , [4] . Th17 induction is supported by interleukin (IL)-1β, IL-6, IL-23 and transforming growth factor-β (TGF-β) [5] , [6] , [7] , cytokines that upregulate and stabilize retinoic acid receptor-related organ receptor (RORγT) and pro-inflammatory function [8] . The cytokine IL-10 preserves gastrointestinal homeostasis [9] . Mice deficient in IL-10 or IL-10Rβ develop spontaneous enterocolitis [10] , [11] . Bi-allelic mutations in IL-10 lead to infantile enterocolitis, polymorphisms in IL-10 are associated with ulcerative colitis and Crohn’s disease, and an association has been further reported between IL-10Rα single-nucleotide polymorphisms (SNPs) and early onset UC [12] , [13] , [14] , [15] . Dynamic interactions between IL-10 and different IL-10 responsive immune cell lineages participate in IBD pathogenesis [16] . Mice with a deletion of IL-10 or its receptor solely in Foxp3 + T cells can develop spontaneous colitis [17] , [18] . The IL-10R-deficient Foxp3 + T cells display decreased IL-10 secretion itself, potentially linking these phenotypes. Further, two recent studies have implicated the IL-10 response by myeloid populations to mucosal homeostasis and colitis susceptibility. Zigmond et al . [19] used a CX3CR1 promoter-directed Cre to selectively delete IL-10Rα. These mice developed spontaneous colitis and implicated IL-10 in the generation of anti-inflammatory CX3CR1 + myeloid cells necessary for colonic homeostasis. Shouval et al . [20] demonstrated that IL-10Rβ −/− Rag2 −/− mice are susceptible to colitis mediated by total CD4 T-cell transfer. The IL-10Rβ deficiency impedes the generation and activity of anti-inflammatory macrophages, and impairs induced Treg (iTreg) generation and Treg function. IL-10-producing myeloid cells have also been shown to prevent the downregulation of Foxp3 in T-cell transfer colitis, indicating a central role for IL-10 in the crosstalk between regulatory T cell and myeloid populations [21] . Implicating IL-10 in T-cell effector function as well, T-cell-specific blockade of IL-10 signalling using a dominant negative IL-10 receptor (IL-10RDN) leads to increased Th17 cells in an anti-CD3 antibody (Ab)-induced model of small intestinal inflammation [22] . Despite the clear role of IL-10 in intestinal homeostasis, pharmacologic administration of IL-10 has not proven effective [23] . Further resolution of the core interactions, responsible cell types, and pertinent mechanisms underlying the activity of IL-10 will be necessary to develop effective interventions targeting this pathway. Here we use the transfer of naive CD4 + CD45RB hi T cells into lymphocyte-deficient strains to analyse how the lineage-specific activities of IL-10 influence the pathologic T-cell response. Transferred naive T cells are activated by microbial flora, provoking Th17-dependent colonic inflammation. Studies using IL-10RDN T cells have indicated that the T-cell IL-10 response does not significantly restrain colitis development after CD45RB hi T-cell transfer [24] . We verify this here using T cells conditionally deficient in the specific receptor for IL-10, IL-10Rα. However, we further show using additional targeted deletion models that IL-10 acts dominantly on macrophages (Mφs) to mediate its inhibitory effects, and define how this occurs through a shift in the cytokine dependency of pathologic effector T cells. We show that IL-10 acts on Mφs to potently suppress IL-1β production through several routes, including the inhibition pro-IL-1β production, caspase-1 activation and IL-1β maturation. This not only modulates colitis, but also transforms the pathologic Th17 response from one that is IL-6-independent and IL-1-dependent to one with an obligate requirement for IL-6. Our findings demonstrate a redundancy in operative Th17 induction pathways during colitis, the critical role of the Mφ response to IL-10 in controlling these pathways, and imply that coordinated therapies targeting redundant cytokines may be required to fully suppress disease. T-cell IL-10 response does not influence colitis development To evaluate lineage-specific effects of IL-10 in T-cell transfer-mediated colitis, we first produced mice with a selective deletion of the specific IL-10 receptor, IL-10Rα, restricted to T cells (IL-10Rα Tdel ) [25] . Colitis was then induced by transferring naive CD4 + CD25 − CD45RB hi T cells from wild-type (WT) or IL-10Rα Tdel mice into Rag1 −/− recipients. Disease magnitude and quality were monitored through changes in body weight, colon histopathology and colonic T cell and T-cell subset (Th1, Th17 and Foxp3 + ) infiltration ( Supplementary Fig. 1 ). No differences were identified between recipients of WT and IL-10Rα Tdel T cells, indicating that IL-10 signalling into the transferred T cells does not modulate colitis severity in this T-cell-dependent model. Mφ response to IL-10 restrains T-cell-mediated colitis We previously demonstrated that macrophage but not dendritic cell (DC) or T-cell IL-10 signalling prominently alleviated inflammation in a distinct T-cell-independent, toxin-induced model of acute colitis, dextran sulfate sodium (DSS) colitis [26] . Recent data have also implicated myeloid cells as regulators of disease severity in T-cell transfer colitis [19] , [20] , [21] . To assess the impact of DC and Mφ-selective deletion of IL-10Rα (IL-10Rα DCdel , IL-10Rα Mdel ) in T-cell transfer colitis, we generated lineage-specific knockouts on a Rag1 −/− background and induced disease. Histologic and clinical disease did not differ between Rag1 −/− and IL-10Rα DCdel Rag1 −/− recipients ( Supplementary Fig. 2a,b ). In contrast, disease was intensified in IL-10Rα Mdel Rag1 −/− mice ( Fig. 1a and Supplementary Fig. 2a,b ). Weight loss was elevated and accelerated, with a mean±s.e.m. decrement at 8 weeks of 19.1±1.1% versus 9.3±1.1% for Rag1 −/− controls ( Fig. 1a ). IL-10Rα Mdel Rag1 −/− colons were shorter than Rag1 −/− controls (8.2±0.3 versus 7.1±0.2 cm, Fig. 1b ). Histopathology in IL-10Rα Mdel Rag1 −/− colons demonstrated increased inflammation, with more extensive cellular infiltrates, submucosal oedema and epithelial erosion ( Fig. 1c ). Total histologic score was 8.3±0.6 and 3.6±0.7 (scale 0–12) for IL-10Rα Mdel Rag1 −/− and Rag1 −/− mice, respectively. Moreover, fewer IL-10Rα Mdel Rag1 −/− mice survived with extended disease times ( Fig. 1d ), and these developed an elevated incidence of rectal prolapse (75% IL-10Rα Mdel Rag1 −/− mice versus 0% Rag1 −/− controls at 12 weeks). 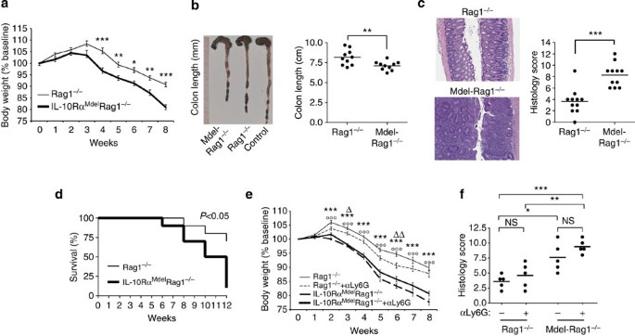Figure 1: Mφ IL-10Rα expression attenuates T-cell-induced colitis. (a) CD4+CD25−CD45RBhiC57BL/6 T cells (5 × 105) were transferred into C57BL/6 Rag1−/−and IL-10RαMdelRag1−/−mice to induce colitis. Mean±1 s.e.m. percent of initial body weight is plotted. *P<0.05; **P<0.01; ***P<0.001 (byt-test). (b) Colons were removed at week 8 and colon length measured from the indicated recipients or mice not receiving T cells (control). (c) Representative photomicrographs and tallied scores for disease parameters from H&E-stained colon sections obtained 8 weeks after naive T-cell transfer. (d) Kaplan–Meier survival curves of Rag1−/−and IL-10RαMdelRag1−/−mice (n=10). (e) Colitis was induced in Rag1−/−and IL-10RαMdelRag1−/−mice with 5 × 105CD4+CD25−CD45RBhiT cells from C57BL/6 mice. Anti-Ly6G or control Ab was administered i.p. 1 day pre-transfer and then weekly to deplete neutrophils. Mean±1 s.e.m. initial body weight is plotted (n=10 per cohort).Δ, Rag1−/−versus Rag1−/−+αLy6G; °, Rag1−/−versus IL-10RαMdelRag1−/−; *, Rag1−/−+αLy6G versus IL-10RαMdelRag1−/−+αLy6G;P<0.05,P<0.01 andP<0.001 for 1, 2 and 3 symbols (by analysis of variance (ANOVA)). No significant difference was seen in IL-10RαMdelRag1−/−versus IL-10RαMdelRag1−/−+αLy6G. (f) Histology scores for 8-week colon from mouse cohorts treated as ine. Data are representative of three independent experiments,n=5–10 per cohort. Figure 1: Mφ IL-10Rα expression attenuates T-cell-induced colitis. ( a ) CD4 + CD25 − CD45RB hi C57BL/6 T cells (5 × 10 5 ) were transferred into C57BL/6 Rag1 −/− and IL-10Rα Mdel Rag1 −/− mice to induce colitis. Mean±1 s.e.m. percent of initial body weight is plotted. * P <0.05; ** P <0.01; *** P <0.001 (by t -test). ( b ) Colons were removed at week 8 and colon length measured from the indicated recipients or mice not receiving T cells (control). ( c ) Representative photomicrographs and tallied scores for disease parameters from H&E-stained colon sections obtained 8 weeks after naive T-cell transfer. ( d ) Kaplan–Meier survival curves of Rag1 −/− and IL-10Rα Mdel Rag1 −/− mice ( n =10). ( e ) Colitis was induced in Rag1 −/− and IL-10Rα Mdel Rag1 −/− mice with 5 × 10 5 CD4 + CD25 − CD45RB hi T cells from C57BL/6 mice. Anti-Ly6G or control Ab was administered i.p. 1 day pre-transfer and then weekly to deplete neutrophils. Mean±1 s.e.m. initial body weight is plotted ( n =10 per cohort). Δ , Rag1 −/− versus Rag1 −/− +αLy6G; °, Rag1 −/− versus IL-10Rα Mdel Rag1 −/− ; *, Rag1 −/− +αLy6G versus IL-10Rα Mdel Rag1 −/− +αLy6G; P <0.05, P <0.01 and P <0.001 for 1, 2 and 3 symbols (by analysis of variance (ANOVA)). No significant difference was seen in IL-10Rα Mdel Rag1 −/− versus IL-10Rα Mdel Rag1 −/− +αLy6G. ( f ) Histology scores for 8-week colon from mouse cohorts treated as in e . Data are representative of three independent experiments, n =5–10 per cohort. Full size image In a recent study, mice deleting IL-10R using a CX3CR1-driven Cre that is expressed by a large proportion of lamina propria macrophages (LPMφs) developed spontaneous colitis. We did not observe overt spontaneous disease in our IL-10Rα Mdel Rag1 −/− mice during the time frame of our assays. To further assess this, cohorts of these and IL-10Rα fl/fl Rag1 −/− controls ( n =10 for each) were aged for 6 months. There was no difference in weight gain, or presence of clinical signs of colitis or other illnesses in either population ( Supplementary Fig. 2c ). Histologic analysis of five aged IL-10Rα Mdel Rag1 −/− mice failed to identify evidence for colitis. Similarly, spontaneous colitis was not observed in 6-month-old IL-10Rα Mdel Rag1 +/+ mice. The protective role of IL-10 in colitis is well established. To determine whether the Mφ-specific response to IL-10 can account for this, we also compared disease in IL-10Rα Mdel Rag1 −/− mice with Rag1 −/− mice harbouring a germline deletion in IL-10Rα (IL-10Rα −/− Rag1 −/− ; Supplementary Fig. 2a,b ). No difference in clinical disease or histopathology was evident in these two recipient lines, implying that IL-10-mediated immunoprotection can largely be accounted for by its Mφ-specific effects. The Lys-M-Cre transgene used to ablate IL-10Rα in the IL-10Rα Mdel Rag1 −/− mice is expressed in granulocytes as well as Mφs [27] . Neutrophils have a modest protective role in T-cell transfer colitis [28] , and loss of IL-10Rα signalling there, rather than in Mφs, may have influenced disease. To isolate the Mφ-specific effect, we depleted neutrophils with specific Ab beginning before T-cell transfer. Neutrophils were undetectable in the peripheral blood from αLy6G Ab but not control Ab-treated animals throughout the experimental interval. In Rag1 −/− recipients, weight loss was mildly increased on some disease days in neutrophil-depleted mice, although no significant difference in histopathology was identified ( Fig. 1e,f ). No significant change in disease severity was apparent with neutrophil depletion in IL-10Rα Mdel Rag1 −/− mice. Further, the prominent disease exacerbation in IL-10Rα Mdel Rag1 −/− compared with Rag1 −/− recipients persisted after neutrophil depletion, indicating that the intensified immunopathology in IL-10Rα Mdel Rag1 −/− mice is primarily attributable to the Mφ rather than granulocyte IL-10 response. Increased numbers and activation of IL-10Rα Mdel Rag1 −/− LPMφs To identify causes of the enhanced IL-10Rα Mdel Rag1 −/− disease, we first analysed LPMφs. LPMφs, typed as CD11b hi CD11c −/lo/mod F4/80 + Ly6G –/lo SiglecF – , were significantly increased in IL-10Rα Mdel Rag1 −/− mice with colitis compared with Rag1 −/− controls ( Fig. 2a ). This population was uniformly CD64 + and predominantly CX3CR1 + , further delineating them as LPMφs [29] , [30] ( Supplementary Fig. 3a ). The cells were further characterized by a uniformly elevated surface expression of activation markers, including CD40, CD80 and CD86 ( Fig. 2b ). Segregation of CD11b + CD64 + CD103 − and CD45 + cells based on Ly6C and class II major histocompatibility complex expression can distinguish pro-inflammatory (Ly6C hi ) and anti-inflammatory (Ly6C lo ) macrophage populations [20] , [30] . Most LPMφs analysed using this alternative gating strategy were phenotypically pro-inflammatory, and the proportions of Ly6C hi and Ly6C lo macrophages did not differ between IL-10Rα Mdel Rag1 −/− mice and Rag1 −/− controls ( Supplementary Fig. 3b ). 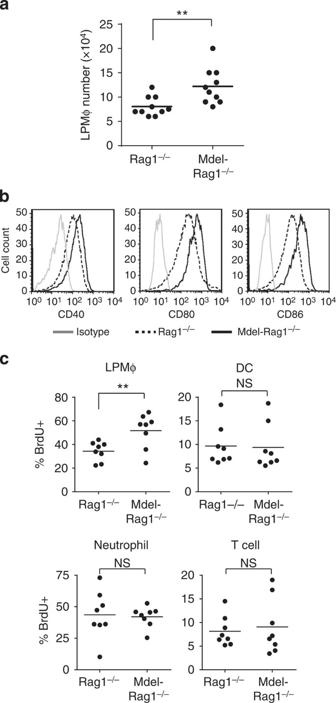Figure 2: Analysis of lamina propria macrophages. (a) Cells were isolated from the large intestine lamina propria of Rag1−/−and IL-10RαMdelRag1−/−mice at week 8 after colitis induction. Absolute numbers of LPMφ (CD11bhiCD11c−/lo/modF4/80+Ly6G–/loSiglecF–) were quantified. (b) Staining of LPMφ gated as above, for CD40, CD80 and CD86. Grey line, isotype control; dashed black line, LPMφs from Rag1−/−mice; solid black line, LPMφs from IL-10RαMdelRag1−/−mice. (c) Rag1−/−and IL-10RαMdelRag1−/−mice received 5 × 105CD4+CD25−CD45RBhiC57BL/6 T cells. After 8 weeks, BrdU was administered i.p. and the mice killed 24 h later. Colon LP cells were isolated and BrdU-positive Mφs, DCs, neutrophils and CD4+T cells measured by intracellular flow cytometry. Data are representative of three independent experiments,n=8–10 per cohort. **P<0.01 (byt-test). Figure 2: Analysis of lamina propria macrophages. ( a ) Cells were isolated from the large intestine lamina propria of Rag1 −/− and IL-10Rα Mdel Rag1 −/− mice at week 8 after colitis induction. Absolute numbers of LPMφ (CD11b hi CD11c −/lo/mod F4/80 + Ly6G –/lo SiglecF – ) were quantified. ( b ) Staining of LPMφ gated as above, for CD40, CD80 and CD86. Grey line, isotype control; dashed black line, LPMφs from Rag1 −/− mice; solid black line, LPMφs from IL-10Rα Mdel Rag1 −/− mice. ( c ) Rag1 −/− and IL-10Rα Mdel Rag1 −/− mice received 5 × 10 5 CD4 + CD25 − CD45RB hi C57BL/6 T cells. After 8 weeks, BrdU was administered i.p. and the mice killed 24 h later. Colon LP cells were isolated and BrdU-positive Mφs, DCs, neutrophils and CD4 + T cells measured by intracellular flow cytometry. Data are representative of three independent experiments, n =8–10 per cohort. ** P <0.01 (by t -test). Full size image The increased IL-10Rα Mdel Rag1 −/− versus Rag1 −/− LPMφ numbers were further associated with an increased proliferation rate, as determined by incorporation of the nucleotide analogue 5-bromodeoxyuridine (BrdU). Unlike for LPMφs, no differences in BrdU incorporation were evident in colonic CD4 T cells, DCs and neutrophils, or in Mφs from other locations ( Fig. 2c ). Therefore, numbers, proliferation and activation state of LPMφs are increased in IL-10Rα Mdel Rag1 −/− mice. Unimpaired IL-10Rα Mdel Rag1 −/− T regulatory response A subset of T cells transferred into Rag1 −/− mice upregulate Foxp3, and IL-10 signalling into Mφs could contribute to the generation and maintenance of these regulatory T cells [21] , [22] . Indeed, recent findings with IL-10Rβ −/− Rag2 −/− mice have identified defective iTreg formation and Treg function. Treg co-transferred with naive T cells even at a 1:1 ratio were incapable of preventing disease [20] . To assess Treg activity here, we quantified Foxp3 + iTreg forming in the lamina propria (LP), mesenteric lymph nodes (MLNs) and spleen of IL-10Rα Mdel Rag1 −/− and control Rag1 −/− colitic mice. No differences were observed ( Fig. 3a ). We next analysed whether sorted Treg transferred into IL-10Rα Mdel Rag1 −/− and Rag1 −/− mice with the induction of colitis could prevent disease. The transferred cells were able to fully suppress disease development in both IL-10Rα Mdel Rag1 −/− and Rag1 −/− recipients, indicating that a macrophage-specific defect in IL-10 response does not overtly have an impact on Treg-suppressive activity in this setting ( Fig. 3b ). Treg transfers led to a more than twofold increase in Treg in the spleens, MLNs and colons of recipient mice, and Treg percentages did not differ between IL-10Rα Mdel Rag1 −/− and Rag1 −/− recipients in any of the locations ( Fig. 3c ). These results indicate that Tregs are able to suppress disease in the absence of a macrophage-specific response to IL-10, and that Treg-specific mechanisms independent of IL-10 actions on macrophages are employed in this system. 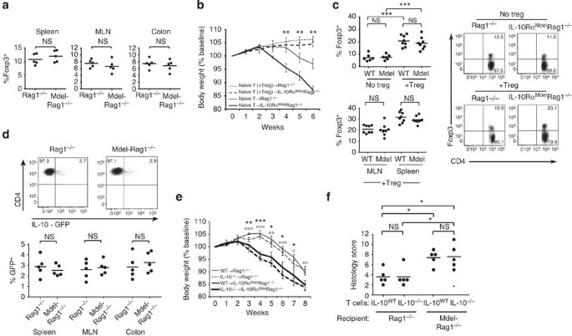Figure 3: T-cell Foxp3 expression and IL-10 production. (a) Colitis was induced in Rag1−/−and IL-10RαMdelRag1−/−mice by the transfer of 5 × 105CD4+CD25−CD45RBhiC57BL/6 T cells. The frequency of Foxp3+Treg cells among CD4+T cells in the spleen, MLN and colon 8 weeks after initial T-cell transfer is plotted. (b) Mice received sorted CD4+CD45RbloFoxp3-YFP+Treg with naive T cells at a 1:1 ratio or naive (CD4+CD45RbhiFoxp3-YFP−)T cells alone, and were monitored for weight loss. **P<0.01 for naive T→Rag1−/−versus naive T→IL-10RαMdelRag1−/−(by ANOVA). Differences were not significant between naive T+Treg→Rag1−/−versus naive T+Treg →IL-10RαMdelRag1−/−cohorts. (c) Splenic, MLN and colonic Foxp3+T cells were identified by flow cytometry in mice receiving or not receiving Treg as inb. Upper left and right plots depict results for colonic Treg. Lower left plot depicts results for MLN and splenic Treg only in mice receiving supplemental Treg. ***P<0.001 (by ANOVA). (d) Similar transfers were performed using CD4+CD25−CD45RBhiT cells from IL-10-GFP donors. Representative dot plots and summary analysis of the frequency of IL-10-GFP+cells among CD4+T cells in the spleen, MLN and colon at 8 weeks is shown. (e) Rag1−/−and IL-10RαMdelRag1−/−mice received 5 × 105CD4+CD25−CD45RBhiT cells from C57BL/6 or IL-10−/−mice. Mean±1 s.e.m. percent initial body weight is plotted. *, WT→Rag1−/−versus WT→IL-10RαMdelRag1−/−; °, IL-10−/−→Rag1−/−versus IL-10−/−→IL-10RαMdelRag1−/−;P<0.05,P<0.01 andP<0.001 for 1, 2 and 3 symbols (by ANOVA). Representative of three independent experiments,n=5 per cohort. (f) Histological scores for colons from the indicated mice at 8 weeks. Figure 3: T-cell Foxp3 expression and IL-10 production. ( a ) Colitis was induced in Rag1 −/− and IL-10Rα Mdel Rag1 −/− mice by the transfer of 5 × 10 5 CD4 + CD25 − CD45RB hi C57BL/6 T cells. The frequency of Foxp3 + Treg cells among CD4 + T cells in the spleen, MLN and colon 8 weeks after initial T-cell transfer is plotted. ( b ) Mice received sorted CD4 + CD45Rb lo Foxp3-YFP + Treg with naive T cells at a 1:1 ratio or naive (CD4 + CD45Rb hi Foxp3-YFP − )T cells alone, and were monitored for weight loss. ** P <0.01 for naive T→Rag1 −/− versus naive T→IL-10Rα Mdel Rag1 −/− (by ANOVA). Differences were not significant between naive T+Treg→Rag1 −/− versus naive T+Treg →IL-10Rα Mdel Rag1 −/− cohorts. ( c ) Splenic, MLN and colonic Foxp3 + T cells were identified by flow cytometry in mice receiving or not receiving Treg as in b . Upper left and right plots depict results for colonic Treg. Lower left plot depicts results for MLN and splenic Treg only in mice receiving supplemental Treg. *** P <0.001 (by ANOVA). ( d ) Similar transfers were performed using CD4 + CD25 − CD45RB hi T cells from IL-10-GFP donors. Representative dot plots and summary analysis of the frequency of IL-10-GFP + cells among CD4 + T cells in the spleen, MLN and colon at 8 weeks is shown. ( e ) Rag1 −/− and IL-10Rα Mdel Rag1 −/− mice received 5 × 10 5 CD4 + CD25 − CD45RB hi T cells from C57BL/6 or IL-10 −/− mice. Mean±1 s.e.m. percent initial body weight is plotted. *, WT→Rag1 −/− versus WT→IL-10Rα Mdel Rag1 −/− ; °, IL-10 −/− →Rag1 −/− versus IL-10 −/− →IL-10Rα Mdel Rag1 −/− ; P <0.05, P <0.01 and P <0.001 for 1, 2 and 3 symbols (by ANOVA). Representative of three independent experiments, n =5 per cohort. ( f ) Histological scores for colons from the indicated mice at 8 weeks. Full size image Alternative regulatory T-cell populations are demarcated by IL-10 production, and IL-10 itself may have an impact on these directly or indirectly. To evaluate this, we induced colitis by transferring naive T cells from IL-10-green fluorescent protein (GFP) knock-in reporter mice. Here too, no differences in population sizes were seen ( Fig. 3d ). To determine whether T-cell IL-10 production was itself functionally dispensable for the differential colitis in IL-10Rα Mdel Rag1 −/− mice, we performed transfers using IL-10 −/− or WT T cells. Disease severity, measured clinically and histologically, was exclusively associated with recipient type. IL-10 production by transferred T cells did not influence disease magnitude clinically or histologically ( Fig. 3e,f ). Therefore, the Mφ IL-10 response does not identifiably have an impact on Treg cell presence. Further, while Mφ response to IL-10 is critical in attenuating disease, T cells are not a significant source of this IL-10 here. Pro-inflammatory cytokine production by IL-10Rα Mdel LPMφs To further evaluate the heightened disease severity in IL-10Rα Mdel Rag1 −/− mice, we measured in whole colons the levels of cytokines implicated in its pathogenesis, including IL-1β, IL-6, TNF (tumour-necrosis factor)-α, monocyte chemoattractant protein (MCP)-1, IL-10, IL-17 and IFN-γ) [31] . With early disease (week 4), IL-1β, IL-6 and MCP-1 were increased in IL-10Rα Mdel Rag1 −/− colon compared with Rag1 −/− controls ( Fig. 4a ). As disease progressed (week 8), the quantity of cytokine produced was altered. Additional elevations in IL-17 and TNF-α were identified at this time. Differences in IL-10 and IFN-γ were not seen. 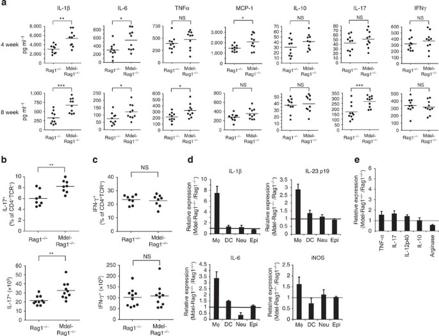Figure 4: Cytokine production by colonic macrophages. (a) Colons from Rag1−/−and IL-10RαMdelRag1−/−mice, 8 weeks after colitis induction, were homogenized and cytokines (IL-1β, IL-6, TNF-α, MCP-1, IL-10, IL-17 and IFN-γ) measured by enzyme-linked immunosorbent assay or multiplex assay. Results from individual mice (circles) and cohort means (lines) are plotted. (b,c) Percent and absolute number of IL-17+and IFN-γ+cells among CD4+T cells from colons of diseased mice (8 weeks). (d) Relative expression of the indicated mRNAs (IL-1β, IL-6, IL-23p19 and iNOS) from LPMφs, DCs, neutrophils and epithelial cells sorted from the colon tissue and measured by qRT–PCR. (e) Relative expression of the indicated mRNAs (TNF-α, IL-17, IL-12p40, IL-10 and arginase) from LPMφs sorted from the colon tissue and measured by qRT–PCR. Data are representative of three independent experiments,n=10 per cohort. *P<0.05; **P<0.01, ***P<0.001 (byt-test). Figure 4: Cytokine production by colonic macrophages. ( a ) Colons from Rag1 −/− and IL-10Rα Mdel Rag1 −/− mice, 8 weeks after colitis induction, were homogenized and cytokines (IL-1β, IL-6, TNF-α, MCP-1, IL-10, IL-17 and IFN-γ) measured by enzyme-linked immunosorbent assay or multiplex assay. Results from individual mice (circles) and cohort means (lines) are plotted. ( b , c ) Percent and absolute number of IL-17 + and IFN-γ + cells among CD4 + T cells from colons of diseased mice (8 weeks). ( d ) Relative expression of the indicated mRNAs (IL-1β, IL-6, IL-23p19 and iNOS) from LPMφs, DCs, neutrophils and epithelial cells sorted from the colon tissue and measured by qRT–PCR. ( e ) Relative expression of the indicated mRNAs (TNF-α, IL-17, IL-12p40, IL-10 and arginase) from LPMφs sorted from the colon tissue and measured by qRT–PCR. Data are representative of three independent experiments, n =10 per cohort. * P <0.05; ** P <0.01, *** P <0.001 (by t -test). Full size image T-cell transfer colitis is associated with colonic infiltration by both Th1 and Th17 cells, and the Th17 response is required for disease development. Our identification of increased colonic IL-6 and IL-1β in IL-10Rα Mdel Rag1 −/− mice, cytokines associated with Th17 induction, coupled with elevated IL-17 but not IFN-γ levels implied an intensification of the Th17 response. To test this, we enumerated IFN-γ- and IL-17-producing T cells in the colonic infiltrate. Significantly increased percents and absolute numbers of CD4 + IL-17A + T cells were identified in IL-10Rα Mdel Rag1 −/− compared with Rag1 −/− colons ( Fig. 4b ). Likewise, after the induction of disease with CD4 + CD25 − CD45RB hi RORγT-GFP reporter T cells, increased GFP + T cells were identified in the colon at 4 and 8 weeks ( Supplementary Fig. 4a ). No differences in CD4 + IFN-γ + T cell quantities were evident ( Fig. 4c ). To more specifically determine whether elevated production of Th17-promoting cytokines was specific to the Mφ population, we sorted colonic CD11b hi CD11c −/lo/mod F4/80 + Ly6G –/lo SiglecF – LPMφs from colitic mice and assayed their cytokine expression profiles by quantitative reverse transcriptase–PCR (qRT–PCR). A particularly prominent elevation in IL-1β production was apparent in IL-10Rα Mdel Rag1 −/− compared with Rag1 −/− LPMφs (mRNA expression ratio: 7.5±1.2). Lesser elevations in IL-6 (3.4±0.5), IL-23 (2.9±0.3) and other pro-inflammatory cytokines were also identified ( Fig. 4d,e ). IL-10 itself was unchanged and a modest decline in arginase with a corresponding increase in iNOS further indicated enhanced pro-inflammatory function of the IL-10Rα Mdel Rag1 −/− LPMφs. For IL-1β, IL-6, IL-23p19 and iNOS, relative expression was compared in sorted colonic LPMφs, DCs, neutrophils and epithelial cells ( Fig. 4d ). Elevated expression was specific to the Mφs, indicating that Mφs are the primary source for the increased Th17-associated cytokines and implying that IL-10 acts directly on these cells to suppress their production. As an alternative gating strategy, we also sorted CD11b + CD64 + CD103 − CD45 + Ly6C hi LPMφs and assessed similarly for IL-1β, IL-6, IL-23, IL-10, iNOS and arginase. These were differentially expressed in a manner paralleling results above ( Supplementary Fig. 4b ). CD163 was additionally assessed as a marker for anti-inflammatory macrophages and found to be similar in the IL-10Rα Mdel Rag1 −/− and control Rag1 −/− populations. Colitis in IL-10Rα Mdel Rag1 −/− mice is Th17-dependent Th17 cells have been shown to be essential to T-cell transfer colitis in Rag1 −/− mice [32] . The elevated colonic inflammation in IL-10Rα Mdel Rag1 −/− mice was correlated with an increased Th17 response, but may also have been mediated by alternative pathologic pathways. To verify a role for Th17 cells, we transferred RORγT −/− T cells into Rag1 −/− and IL-10Rα Mdel Rag1 −/− recipients ( Supplementary Fig. 5 ). RORγT, and hence Th17 cells, proved essential for colitis in both recipient types. Colitis is IL-6-independent in IL-10Rα Mdel Rag1 −/− mice Although IL-6 is well established as a key inducer of Th17 cells, its isolated role in fostering the Th17 response fundamental to T-cell transfer colitis has not been addressed. The increased IL-6 in IL-10Rα Mdel Rag1 −/− mice might have driven the increased immunopathology there. To assess this, we induced colitis by transfers of IL-6Rα −/− or WT naive T cells into IL-10Rα Mdel Rag1 −/− and Rag1 −/− recipients. IL-6Rα −/− T cells were ineffective in inducing disease in Rag1 −/− mice ( Fig. 5a,b ). Mice gained weight after T-cell transfer and histologic lesions were mild. In contrast, IL-6Rα −/− and WT T cells proved equipotent in mediating severe clinical disease in IL-10Rα Mdel Rag1 −/− recipients. Although there was a trend towards modestly diminished histologic severity after IL-6Rα −/− transfer, this was not significant. Thus, the Mφ response to IL-10 creates a dependency for IL-6 in disease pathogenesis. 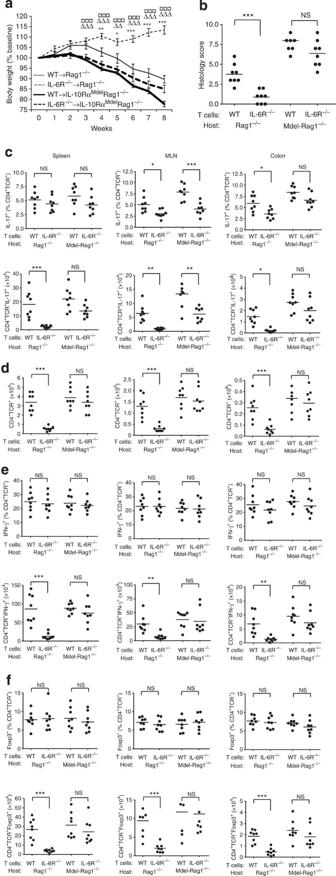Figure 5: Role of T-cell IL-6 response in colitis development in Rag1−/−and IL-10RαMdelRag1−/−mice. Colitis was induced in Rag1−/−and IL-10RαMdelRag1−/−mice by the transfer of 5 × 105C57BL/6 or IL-6Rα−/−CD4+CD25−CD45RBhiT cells. Mice were killed after 8 weeks. (a) Representative weight curves, mean±1 s.e.m., are plotted. *, WT→Rag1−/−versus IL-6Rα−/−→Rag1−/−;Δ, WT→Rag1−/−versus WT→IL-10RαMdelRag1−/−;□, IL-6Rα−/−→Rag1−/−versus IL-6Rα−/−→IL-10RαMdelRag1−/−;P<0.05,P<0.01 andP<0.001 for 1, 2 and 3 symbols (by ANOVA). No significant differences were observed for WT→IL-10RαMdelRag1−/−versus IL-6Rα−/−→IL-10RαMdelRag1−/−. (b) Histologic scores for colons analysed at 8 week. (c) Percent and absolute number of IL-17+cells among CD4+T cells in the spleen, MLN and colon. (d) Absolute numbers of CD4+T cells. (e) Percent and absolute number of IFN-γ+cells among CD4+T cells. (f) Percent and absolute number of Foxp3+Treg cells among CD4+T cells. *P<0.05; **P<0.01; ***P<0.001 (byt-test). Data are representative of three independent experiments,n=8 per cohort. Figure 5: Role of T-cell IL-6 response in colitis development in Rag1 −/− and IL-10Rα Mdel Rag1 −/− mice. Colitis was induced in Rag1 −/− and IL-10Rα Mdel Rag1 −/− mice by the transfer of 5 × 10 5 C57BL/6 or IL-6Rα −/− CD4 + CD25 − CD45RB hi T cells. Mice were killed after 8 weeks. ( a ) Representative weight curves, mean±1 s.e.m., are plotted. *, WT→Rag1 −/− versus IL-6Rα −/− →Rag1 −/− ; Δ , WT→Rag1 −/− versus WT→IL-10Rα Mdel Rag1 −/− ; □ , IL-6Rα −/− →Rag1 −/− versus IL-6Rα −/− →IL-10Rα Mdel Rag1 −/− ; P <0.05, P <0.01 and P <0.001 for 1, 2 and 3 symbols (by ANOVA). No significant differences were observed for WT→IL-10Rα Mdel Rag1 −/− versus IL-6Rα −/− →IL-10Rα Mdel Rag1 −/− . ( b ) Histologic scores for colons analysed at 8 week. ( c ) Percent and absolute number of IL-17 + cells among CD4 + T cells in the spleen, MLN and colon. ( d ) Absolute numbers of CD4 + T cells. ( e ) Percent and absolute number of IFN-γ + cells among CD4 + T cells. ( f ) Percent and absolute number of Foxp3 + Treg cells among CD4 + T cells. * P <0.05; ** P <0.01; *** P <0.001 (by t -test). Data are representative of three independent experiments, n =8 per cohort. Full size image To better understand this, we analysed the T-cell responses leading to colonic injury. Th17 cell percentages among CD4 + TCR + T cells were reduced in the MLNs of mice receiving IL-6Rα −/− T cells ( Fig. 5c ). This was true for both IL-10Rα Mdel Rag1 −/− and Rag1 −/− mice. Thus, IL-6Rα signalling supports but is not essential for Th17 formation in the MLNs of both of these recipient lines. In the colon, the representation of Th17 cells was significantly decreased in Rag1 −/− but not IL-10Rα Mdel Rag1 −/− recipients. This indicates a relative expansion of Th17 cells at the site of autoimmune inflammation specifically in IL-10Rα Mdel Rag1 −/− mice. Absolute numbers of Th17 cells in all organs sampled dramatically differed between Rag1 −/− and IL-10Rα Mdel Rag1 −/− recipients of IL-6Rα −/− T cells. Few Th17 cells were present in the spleens, MLNs and colons of Rag1 −/− recipients, whereas large numbers were present in IL-10Rα Mdel Rag1 −/− recipients ( Fig. 5c ). This difference reflected a pervasive decrease in total T-cell number with the IL-6Rα −/− →Rag1 −/− transfers ( Fig. 5d ). Therefore, IL-6 is broadly necessary for T-cell expansion and colitis in Rag1 −/− but dispensable in IL-10Rα Mdel Rag1 −/− mice. Actions of IL-10 on Mφs generate an IL-6 requirement for autoinflammatory disease and robust T-cell expansion. In contrast to Th17 development, no differences were identified in the proportions of Th1 or Foxp3 + CD4 + T cells in any of the transfer combinations tested, indicating that T-cell IL-6 and Mφ IL-10 responses do not similarly skew these maturation pathways ( Fig. 5e,f ). However, absolute numbers of Th1 and Foxp3 + cells were diminished in the IL-6Rα −/− →Rag1 −/− combination, again reflecting the impaired T-cell expansion in the absence of disease development. IL-1 response is required for IL-10Rα Mdel Rag1 −/− colitis IL-1β plays an essential role in the steady-state development of intestinal Th17 cells in healthy mice [33] and further promotes the Th17 response during colitis [34] . Considering this, the lack of a requirement for IL-6 in IL-10Rα Mdel Rag1 −/− mice ( Fig. 5a,b ), and the dramatically elevated IL-1β expression in IL-10Rα Mdel Rag1 −/− LPMφs ( Fig. 4 ), we hypothesized that IL-1β plays a pathologic role in IL-10Rα Mdel Rag1 −/− mice that is able to supersede the IL-6 requirement for colitis. To test the impact of IL-1, we induced colitis by transferring IL-1R −/− T cells into IL-10Rα Mdel Rag1 −/− and Rag1 −/− recipients. IL-1R −/− T-cell transfers into Rag1 −/− mice did not lead to the virtually complete disease protection seen after IL-6Rα −/− T-cell transfers. However, IL-1R −/− →Rag1 −/− transfers did show diminished clinical and histologic measures of colitis compared with control WT T-cell transfers ( Fig. 6a,b ). IL-1R −/− T cells also provoked significantly milder disease than WT T cells in IL-10Rα Mdel Rag1 −/− recipients ( Fig. 6a,b ). This contrasts with IL-6Rα −/− T cells, which did not detectably alter disease severity. Therefore, while T-cell IL-6 responsiveness is clinically important only in Rag1 −/− colitis, T-cell IL-1 response modulates both Rag1 −/− and IL-10Rα Mdel Rag1 −/− disease. 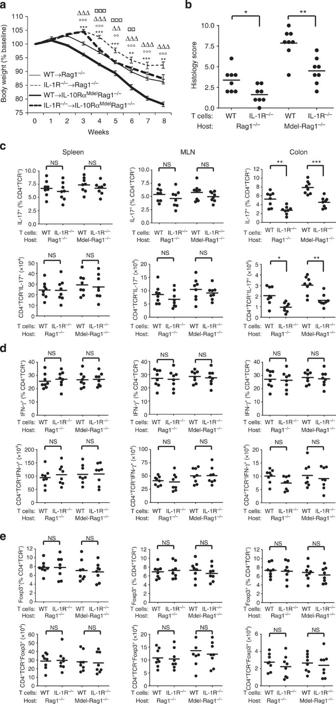Figure 6: Role of T-cell IL-1 response in colitis development in Rag1−/−and IL-10RαMdelRag1−/−mice. Colitis was induced in Rag1−/−and IL-10RαMdelRag1−/−mice by the transfer of 5 × 105C57BL/6 or IL-1R−/−CD4+CD25−CD45RBhiT cells. Mice were killed after 8 weeks. (a) Representative weight curves, mean±1 s.e.m., are plotted. *, WT→Rag1−/−versus IL-1R−/−→Rag1−/−; °, WT→IL-10RαMdelRag1−/−versus IL-1R−/−→ IL-10RαMdelRag1−/−;Δ, WT→Rag1−/−versus WT→IL-10RαMdelRag1−/−;□, IL-1R−/−→Rag1−/−versus IL-1R−/−→IL-10RαMdelRag1−/−;P<0.01 andP<0.001 for 2 and 3 symbols (by ANOVA). (b) Histologic scores for colons analysed at 8 weeks. (c) Percent and absolute number of IL-17+cells among CD4+T cells in the spleen, MLN and colon. (d) Percent and absolute number of IFN-γ+cells among CD4+T cells. (e) Percent and absolute number of Foxp3+Treg cells among CD4+T cells. *P<0.05; **P<0.01; ***P<0.001 (byt-test). Data are representative of three independent experiments,n=8 per cohort. Figure 6: Role of T-cell IL-1 response in colitis development in Rag1 −/− and IL-10Rα Mdel Rag1 −/− mice. Colitis was induced in Rag1 −/− and IL-10Rα Mdel Rag1 −/− mice by the transfer of 5 × 10 5 C57BL/6 or IL-1R −/− CD4 + CD25 − CD45RB hi T cells. Mice were killed after 8 weeks. ( a ) Representative weight curves, mean±1 s.e.m., are plotted. *, WT→Rag1 −/− versus IL-1R −/− →Rag1 −/− ; °, WT→IL-10Rα Mdel Rag1 −/− versus IL-1R −/− → IL-10Rα Mdel Rag1 −/− ; Δ , WT→Rag1 −/− versus WT→IL-10Rα Mdel Rag1 −/− ; □ , IL-1R −/− →Rag1 −/− versus IL-1R −/− →IL-10Rα Mdel Rag1 −/− ; P <0.01 and P <0.001 for 2 and 3 symbols (by ANOVA). ( b ) Histologic scores for colons analysed at 8 weeks. ( c ) Percent and absolute number of IL-17 + cells among CD4 + T cells in the spleen, MLN and colon. ( d ) Percent and absolute number of IFN-γ + cells among CD4 + T cells. ( e ) Percent and absolute number of Foxp3 + Treg cells among CD4 + T cells. * P <0.05; ** P <0.01; *** P <0.001 (by t -test). Data are representative of three independent experiments, n =8 per cohort. Full size image We performed similar analyses of the impact on T-cell responses after IL-1R −/− transfers as for the IL-6Rα −/− transfers above. Whereas a decreased percent and absolute number of Th17 cells was seen in the MLNs, a site of T-cell priming, after IL-6Rα −/− transfers ( Fig. 5c ), no differences in the MLNs were seen for IL-10Rα Mdel Rag1 −/− or Rag1 −/− recipients receiving IL-1R −/− compared with WT T cells ( Fig. 6c ). However, substantially diminished proportions and absolute numbers of Th17 cells were seen in the colons of mice receiving IL-1R −/− T cells. The actions of IL-1 were specific to Th17 effectors; no differences were identified in Th1 and Foxp3 + Treg populations ( Fig. 6d,e ). This indicates that there is a selective defect in the Th17 response in the colon. T-cell IL-1 but not IL-6 response in IL-10Rα Mdel Rag1 −/− mice promotes colonic inflammation by supporting Th17 cells at the site of autoinflammatory disease. In Rag1 −/− mice, where IL-10 suppresses LPMφ IL-1β production, IL-6 plays a more critical role. Il-10 inhibits pro-IL-1β production and maturation Our data indicated that IL-1β, increased in the colon of IL-10Rα Mdel mice, supports the pathologic Th17 response mediating colitis. IL-10 inhibits this IL-1β production, thereby attenuating disease. To determine whether IL-1β protein in the colon is primarily produced by LPMφs, we used immunohistochemistry to colocalize IL-1β and CD11b in colon sections from diseased IL-10Rα Mdel Rag1 −/− and Rag1 −/− mice ( Supplementary Fig. 6a ). This demonstrated that IL-1β is largely associated with the CD11b + population. IL-1β is generated from an inactive cytosolic precursor (pro-IL-1β). Caspase-1 cleaves pro-IL-1β, converting it into its active form, which is then released from the cell [35] . Caspase-1, in turn, is activated by inflammasome stimulation [36] . To better evaluate the impact of IL-10 signalling on IL-1β production by LPMφs, we first quantified pro-IL-1β levels by flow cytometry in gated CD11b hi CD11c −/lo/mod F4/80 + Ly6G –/lo SiglecF – Mφs. This demonstrated a 1.7-fold elevation in the percent of LPMφs expressing pro-IL-1β in the colons of diseased IL-10Rα Mdel Rag1 −/− compared with Rag1 −/− mice (mean±s.d. : 84.6±6.0% versus 48.6±8.4%; Fig. 7a ). Further, the mean fluorescence intensity of positive cells from IL-10Rα Mdel Rag1 −/− mice was nearly twofold greater than that from control mice (131.4±9.3 versus 76.6±5.7). In contrast to the colons of diseased mice, pro-IL-1β levels were low to undetectable in MLN and bone marrow macrophages, and levels did not differ between IL-10Rα Mdel Rag1 −/− mice and Rag1 −/− controls. Differences in pro-IL-1β were also not apparent in mice in which disease was not induced ( Supplementary Fig. 6b ). 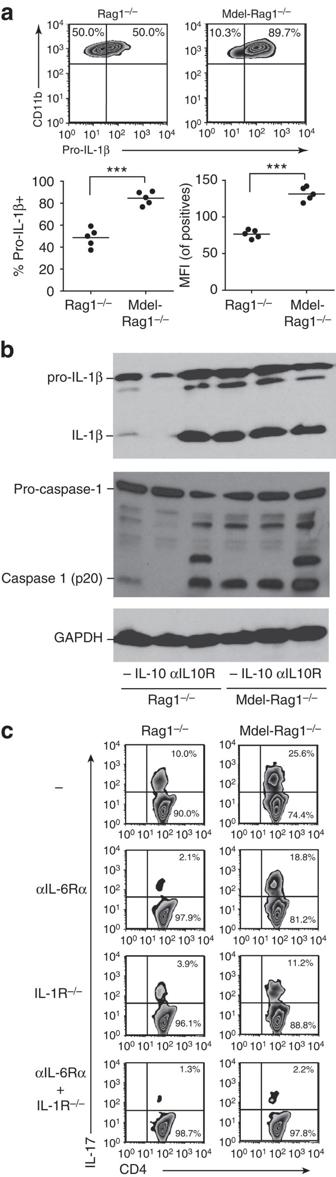Figure 7: IL-10 inhibition of Mφ inflammasome activity and IL-1β production. (a) Colitis was induced in Rag1−/−and IL-10RαMdelRag1−/−mice by the transfer of 5 × 105CD4+CD25−CD45RBhiT cells from WT mice. After 8 weeks, LPMφ pro-IL-1β expression was assessed by intracellular staining. Percent of Mφs expressing pro-IL-1β and the mean fluorescence intensity (MFI) of positive cells are plotted. Data are representative of three independent experiments,n=5 per cohort. ***P<0.001 (byt-test). (b) Rag1−/−and IL-10RαMdelRag1−/−BMDMs were pretreated with recombinant murine IL-10 or blocking anti-IL-10Rα Ab for 4 h before the addition of LPS for 12 h and ATP for the final 30 min. Lysates were immunoblotted for IL-1β, caspase-1 and GAPDH. (c) Naive CD4+T cells from WT or IL-1R−/−mice and LPMφs from colitic Rag1−/−and IL-10RαMdelRag1−/−mice were purified by flow cytometric sorting. The T cells were stimulated with anti-CD3 and anti-CD28 in the presence of anti-IL-4, anti-IFN-γ and TGF-β. LPMφs and T-cell source, and the addition of blocking anti-IL-6R Ab are indicated. After 4 days, IL-17-producing cells were analysed by intracellular staining. Figure 7: IL-10 inhibition of Mφ inflammasome activity and IL-1β production. ( a ) Colitis was induced in Rag1 −/− and IL-10Rα Mdel Rag1 −/− mice by the transfer of 5 × 10 5 CD4 + CD25 − CD45RB hi T cells from WT mice. After 8 weeks, LPMφ pro-IL-1β expression was assessed by intracellular staining. Percent of Mφs expressing pro-IL-1β and the mean fluorescence intensity (MFI) of positive cells are plotted. Data are representative of three independent experiments, n =5 per cohort. *** P <0.001 (by t -test). ( b ) Rag1 −/− and IL-10Rα Mdel Rag1 −/− BMDMs were pretreated with recombinant murine IL-10 or blocking anti-IL-10Rα Ab for 4 h before the addition of LPS for 12 h and ATP for the final 30 min. Lysates were immunoblotted for IL-1β, caspase-1 and GAPDH. ( c ) Naive CD4 + T cells from WT or IL-1R −/− mice and LPMφs from colitic Rag1 −/− and IL-10Rα Mdel Rag1 −/− mice were purified by flow cytometric sorting. The T cells were stimulated with anti-CD3 and anti-CD28 in the presence of anti-IL-4, anti-IFN-γ and TGF-β. LPMφs and T-cell source, and the addition of blocking anti-IL-6R Ab are indicated. After 4 days, IL-17-producing cells were analysed by intracellular staining. Full size image We verified that pro-IL-1β was directly regulated in Mφ by IL-10, analysing its production in cultured and lipopolysaccharide (LPS) and ATP-stimulated Mφ by western blot analysis, and simultaneously assessing for mature IL-1β formation ( Fig. 7b and Supplementary Fig. 7 ). Substantially lower amounts of both pro-IL-1β and IL-1β were present in cultures of Rag1 −/− than IL-10Rα Mdel Rag1 −/− Mφ. After treatment with IL-10, pro-IL-β was diminished and mature IL-1β undetectable in Rag1 −/− cultures, while this manipulation had no effect on IL-10Rα Mdel Rag1 −/− -derived Mφs. In contrast, treatment with blocking anti-IL-10R antibody elevated Rag1 −/− pro-IL-1β and IL-1β levels to those seen with IL-10Rα Mdel Rag1 −/− Mφs. The complete suppression of IL-1β maturation by IL-10 suggested that Mφ IL-10R signalling also suppressed caspase-1 activation. To test this, we assessed for caspase-1 cleavage to its activated form. LPS and ATP stimulation of Rag1 −/− Mφs led to a modest increase in activated caspase-1 (p20, Fig. 7b and Supplementary Fig. 7 ). Pre-treatment of Rag1 −/− Mφs with IL-10, however, abrogated this induction. In contrast, pre-treatment with anti-IL-10Rα Ab markedly increased activated caspase-1, indicating that autocrine IL-10 normally restrains caspase-1 activation. In the IL-10Rα Mdel Rag1 −/− Mφs, p20 formation was similarly increased regardless of IL-10 or anti-IL-10Rα Ab treatment. To determine whether increased IL-1 and IL-6 from LPMφs can also directly have an impact on Th17 cell maturation, we sorted LPMφs from diseased IL-10Rα Mdel Rag1 −/− and control Rag1 −/− mice, and co-cultured them with naive T cells in the presence of added TGFβ but not IL-6. Some Th17s formed in the presence of Rag1 −/− LPMφs; however, this was markedly elevated with IL-10Rα Mdel Rag1 −/− LPMφs ( Fig. 7c ). Addition of αIL-6Rα blocking antibody largely abrogated Th17 formation with Rag1 −/− LPMφs. However, consistent with our in vivo findings after IL-6R −/− T-cell transfer, this effect was modest with IL-10Rα Mdel Rag1 −/− -derived LPMφs. Blocking IL-1 signalling led to more substantial inhibition of Th17 development in IL-10Rα Mdel Rag1 −/− -derived LPMφs and inhibition of signalling by both cytokines essentially abrogated Th17 formation. Therefore, IL-10 can act on LPMφs to directly impair their support of Th17 production. This occurs through the downregulation of IL-1 and to a lesser extent IL-6. Anti-inflammatory signals of IL-10 maintain intestinal homeostasis. Yet, the essential targets and mechanisms of IL-10 action are incompletely understood. Recent data have provided support for a myeloid response to IL-10 in restraining colonic inflammation, and indicated a critical role for IL-10 in the production of anti-inflammatory LPMφs that are essential for maintaining immune homeostasis [19] , [20] . We demonstrate here that Mφs are the primary targets of IL-10, limiting colitis after naive T-cell transfer into immunodeficient mice. We further identify how the macrophage-specific response to IL-10 skews the production and expansion of pathologic T cells, thereby promoting disease exacerbation. Colitis is Th17-dependent regardless of Mφ IL-10 response. However, we show that IL-10 converts the disease from one that is independent of the Th17 inducing cytokine IL-6 to one that is highly dependent. In Rag1 −/− recipients of CD4 + CD45RB hi T cells, T-cell responsiveness to IL-6 is necessary for Th17 formation and colitis development. However, in IL-10Rα Mdel Rag1 −/− recipients of IL-6Rα −/− T cells, a strong Th17 amplification occurs. Colitis develops that is clinically indistinguishable from that in recipients of IL-6Rα WT T cells. Our results further indicate that the Mφ response to IL-10 downmodulates multiple pro-inflammatory cytokines in the colon, but its impact on IL-1β, recently documented to regulate Th17 formation during colitis [34] , appears paramount. IL-10 therefore shifts the cytokine requirements for the Th17 response. In the absence of IL-10, redundancy between IL-1β and IL-6 supports persistent colitis. Implicitly, although monotherapy with anti-IL-6 may be promising, tandem inhibition of the IL-1 pathway may be necessary for optimal suppression of the Th17 response in IBD, particularly where IL-10 signalling is attenuated. Previous studies have indicated a role for IL-1β in promoting Th17 development both in humans and mice [34] , [37] , [38] . IL-1β levels in IL-10 −/− mice with colitis are elevated [39] and we extend this finding here to show that a Mφ-selective deficit in IL-10 response is sufficient for this. Prior in vitro findings have also indicated that IL-1β synergizes with IL-23 to promote Th17 expansion [7] , and we did observe increased IL-23 along with IL-1β production by IL-10Rα-deficient macrophages. Although we and others have identified an essential role for RORγT + Th17 cells in colitis and elevated Th17 cells and/or cytokines have been observed in patients with IBD, the actual role of IL-17 itself is controversial and in a randomized control trial anti-IL-17A proved ineffective in Crohn’s disease [40] . Identifying effector mechanisms responsible for Th17-mediated immunopathology during colitis will be important as new therapeutic strategies are developed. Zigmond et al . [19] recently found that mice with a CX3CR1-restricted IL-10Rα deficiency develop spontaneous colitis. This was hypothesized to be mediated by defective macrophage regulation by IL-10. Our findings are consistent with this and with a unique defining role for macrophages in colitis susceptibility. CX3CR1 is also expressed by DCs [41] and monocytes [42] , and by using IL-10Rα DCdel Rag1 −/− , IL-10Rα Mdel Rag1 −/− , IL-10Rα −/− Rag1 −/− and neutrophil-specific depleted mice, our findings support a dominant role for IL-10 action on macrophages in colitis development. This identification of Mφ as a key target of IL-10 is consistent with a recently published report showing that ATP derived from commensal bacteria promotes Th17 differentiation through a subset of CD11c −/low LP cells [43] . Unlike Zigmond et al ., we did not observe spontaneous autoimmunity in our animals. Differences in microflora, and particularly the presence of Helicobacter spp., may account for this. Our colony is maintained under helicobacter-free conditions, whereas Zigmond et al . report the presence of Helicobacter . Consistently, helicobacter-free IL-10-deficient mice are protected from spontaneous disease [44] . Alternatively, differences in the subsets of Mφs expressing the CX3CR1 versus Lys-M promoters may distinguish spontaneous disease susceptibility in our two systems, and this needs to be further explored. Shouval et al . [20] recently identified a prominent role for IL-10Rβ signalling into myeloid cells in suppressing colitis development. A significant diminution of the Foxp3 + regulatory T-cell response was seen. We did not identify a discernible effect of Mφ IL-10Rα deficiency on iTreg development or transferred nTreg function. This will need resolution. IL-10Rβ is also utilized by IL-22, IL-26 and IFN-λ, which might explain the differences. Alternatively, cell types besides Lys-M + macrophages may provide critical signals supporting Treg formation and maintenance, and IL-10 may be necessary for this. Regardless of these differences, Shouval et al . [20] demonstrated a strongly pro-inflammatory phenotype of IL-10Rβ −/− bone marrow-derived macrophage (BMDM), and extended this to Mφs from IL-10R-deficient patients, implying that these regulatory mechanics are translatable to human IBD. Cumulatively, these data provide strong evidence for macrophage as the critical target of IL-10, and assert several mechanisms through which this occurs. After transfers of IL-6Rα-deficient T cells, we identified a decreased percent of Th17 cells in the MLN but not in the colon of IL-10Rα Mdel Rag1 −/− recipients. This may imply that Th17 cells primed in the MLN are amplified by IL-1β in the colon. However, the site(s) of priming of the Th17 response in colitis is not defined, and it is possible that additional priming occurs within the gut-associated lymphoid tissue itself. In this regards, we show that isolated LPMφs from IL-10Rα Mdel Rag1 −/− mice have an enhanced ability to support Th17 development from naive T cells. Hence, although without being able to track the initial site of pathologic T-cell development we cannot distinguish whether IL-1β in our system is acting at priming or expansion of Th17 cells, increased colonic Mφ IL-1β production can support either or both of these mechanisms. Our results here are consistent with data demonstrating that IL-10 acts via STAT3 to suppress pro-IL-1β production [45] . Moreover, we extend these findings, showing that IL-10 further inhibits caspase-1 activity. Caspase-1 is activated through inflammasome-induced oligomerization and autocatalytic cleavage, and it will be important to identify the precise site at which IL-10 acts within the inflammasome cascade. Although our study specifically interrogates the IL-10 response during colitis, its implications may extend beyond this. IL-1β also promotes the Th17 response in Helicobacter hepaticus colitis [34] . Administration of rIL-1-β selectively induced Th17 cells in the steady-state intestinal environment [33] . High levels of IL-1β are associated with an amplified Th17 response in autoimmune rheumatoid arthritis (RA) and experimental autoimmune encephalomyelitis (EAE) models [46] , [47] , [48] . These effects of IL-1β on Th17 cells may be similarly IL-10- and Mφ-dependent, and this can be assessed using the conditional knockout mice we have developed. Our results, as those using a Tg DN IL-10R [24] , do not support transferred naive T cells as a significant target of IL-10 in this model. This does not indicate that IL-10 is not a significant T-cell regulator. The effects of IL-10 on T cells is complex, and is system- and T-cell subset-dependent. Thus, the Treg response to IL-10 was found to sustain Treg in colitis, and mice with a Treg-selective deletion of IL-10R developed spontaneous colitis [18] , [21] . Likewise, we have identified direct effects of IL-10 on T cells in regulating myelin-specific responses during experimental autoimmune encephalomyelitis [25] . It will also be important to identify the source of IL-10 relevant to Mφ targets. Our findings here and those of others indicate that neither effector nor the adaptive regulatory T cells that form after naive T-cell-transfer are relevant sources [49] . In contrast, purified and adoptively transferred IL-10 −/− Tregs were seen to be less potent than WT Tregs in preventing and treating established colitis, indicating that Treg IL-10 is significant in some circumstances. However, Tregs only account for a portion of IL-10’s effects [49] , [50] , [51] . The absence of a physiologically relevant T-cell IL-10 source here may suggest a myeloid source. Mφ themselves are strong IL-10 producers and autocrine IL-10 signalling may well provide necessary signals that prevent overzealous Mφ reactions. Indeed, we identified substantial IL-10-mediated autoregulation of pro-IL-1β production and caspase-1 activation in cultured Mφ ( Fig. 7 ). In contrast, Zigmond et al . [19] found no role for CX3CR1 + macrophage-produced IL-10 in the spontaneous colitis that they observed, potentially implying that multiple sources may be relevant. In summary, we show that the Mφ response to IL-10 is critical for Th17 development during colitis. Further, the suppression of IL-10 suppression of pro-inflammatory cytokine production does not obviate the essential role for Th17 cells but does shift the cytokine requirements for that response from one primarily governed through IL-1β to one that is IL-6-dependent. Mice We previously produced and verified correct targeting of IL-10Rα fl/fl mice and lineage-specific IL-10Rα deletions on a C57BL/6 background as described in prior publications [25] , [26] . These were bred with B6.129S7-Rag1 tm1Mom /J mice. B6.129P2-IL-10 tm1Cgn /J, B6.129P2-Rorc tm1Litt /J, B6.129S7-Il1r1 tm1mx /J, B6.129(Cg)- Foxp3 tm4(YFP/cre)Ayr /J and B6;SJL-Il6Rα tm1.1Drew /J mice were obtained from The Jackson Laboratories. Colonies were maintained under spf, including detectable Helicobacter spp .-free, conditions. Mice of either sex were between 8 and 12 weeks of age at the time of study, and paired between experimental and control groups. Experimental protocols were approved by the St Jude Animal Care and Use Committee. Induction of colitis Flow cytometrically sorted CD4 + CD25 − CD45RB hi T cells (5 × 10 5 per mouse) derived from pooled splenocytes and lymph node cells of indicated mice were transferred intravenously (i.v.) into Rag1 −/− or IL-10Rα Mdel Rag1 −/− mice. Body weight was monitored on a weekly basis. For neutrophil depletion studies, 1 mg anti-Ly6G mAb 1A8 (Bio-X-Cell) or control IgG [26] was administered per mouse intraperitoneally (i.p.) 1 day before cell transfer and weekly thereafter. Depletion was confirmed by flow cytometry. For analyses of Treg-mediated disease suppression, splenocytes from Foxp3-YFP reporter mice were collected and naive T cells, defined as CD4 + CD45RB hi YFP − , and Treg cells, defined as CD4 + CD45RB low YFP + , sorted. Purity after sorting was >99%. Age-matched Rag1 −/− mice or IL-10Rα Mdel Rag1 −/− mice received 2 × 10 5 naive T cells with or without Treg cells at a 1:1 ratio i.v. Histology Colons were stained with haematoxylin and eosin. Three independent sections were assessed per mouse by a blinded reviewer. Inflammation scoring is as follows: 0, no or occasional inflammatory cells in the LP; 1, increased LP inflammatory cells; 2, confluence of inflammatory cells extending into the submucosa; and 3, transmural infiltrate extension of the infiltrate. Ulceration scoring is as follows: 0, no ulceration; 1, mild (one to two ulcers per 40 crypts analysed); 2, moderate (three to four ulcers); and 3, severe (more than four ulcers). Hyperplasia scoring is as follows: 0, normal; 1, crypts up to twice normal thickness with normal epithelium; 2, crypts more than two times normal thickness, hyperchromatic epithelium; reduced goblet cells, scattered arborization; 3, Crypts more than three times normal thickness, marked hyperchromasia, few to no goblet cells, high mitotic index, frequent arborization. Disease area scoring: 0, 0–5% involvement; 1, 5–30%; 2, 30–70%; 3, >70%. Total score is the sum of individual scores. Cytokine levels Frozen colon samples were homogenized in ice-cold PBS containing 1% NP-40 and complete protease inhibitor cocktail (Roche). Cytokines and chemokines were measured by Luminex (Bio-Rad) or enzyme-linked immunosorbent assay (R&D Systems). LP cell isolation LP cells were isolated using a modification of a previously described protocol [26] . Large intestines were carefully excised, mesentery and fat removed and intestines were then opened longitudinally, rinsed in HBSS and cut into 1-cm pieces. Colon segments were vigorously shaken twice in medium with 1 mM EDTA (Sigma-Aldrich) for 20 min at 37 °C, and suspended cells collected and filtered through a cell strainer. Tissue was further minced and incubated at 37 °C for 1 h in medium with 1 mM collagenase type IV (Sigma-Aldrich) and 40 U ml −1 DNase I (Roche) with agitation. Cells were filtered, washed and isolated over a percoll step gradient. Cytokine PCR Total RNA was isolated from sorted LPMφs using the RNeasy mini kit (Qiagen), and cDNA synthesized using superscript III and oligo (dT) primers (Invitrogen). Expression levels of were normalized to HPRT (Δ C t ) and compared with littermate controls using the ΔΔ C t method [52] . Primer sequences are: TGF-β: F, 5′- CACAGTACAGCAAGGTCCTTGC -3′; R, 5′- AGTAGACGATGGGCAGTGGCT -3′; IL-12p35: F, 5′- ATGACCCTGTGCCTTGGTAG -3′; R, 5′- GATTCTGAAGTGCTGCGTTG -3′; IL-23p19: F, 5′- AGCGGGACATATGAATCTACTAAGAGA -3′; R, 5′- GTCCTAGTAGGGAGGTGTGAAGTT -3′; IL-12p40: F, 5′- GACCATCACTGTCAAAGAGTTTCTAGAT -3′; R, 5′- AGGAAAGTCTTGTTTTTGAAATTTTTTAA -3′; IL-1β: F, 5′- GATCCACACTCTCCAGCTGCA -3′; R, 5′- CAACCAACAAGTGATATTCTCCATG -3′; IL-10: F, 5′- GTGAAAATAAGAGCAAGGCAGTG -3′; R, 5′- ATTCATGGCCTTGTAGACACC -3′; TNF-α: F, 5′- AATGGCCTCCCTCTCATCAGT -3′; R, 5′- CTACAGGCTTGTCACTCGAA -3′; iNOS: F, 5′- TGACGGCAAACATGACTTCAG -3′; R, 5′- GCCATCGGGCATCTGGTA -3′; IL-6: F, 5′- TATGAAGTTCCTCTCTGCAAGAGA -3′; R, 5′- TAGGGAAGGCCGTGGTT -3′; Arginase: F, 5′- TCACTTTCCACCACCTCTTGAY -3′; R, 5′- TCTCCACCGCCTCACGACTC -3′; IL-17A: F, 5′- GCTCCAGAAGGCCCTCAG -3′, R, 5′- CTTTCCCTCCGCATTGACA -3′; CD163: F, 5′- CCTTGGAAACAGAGACAGGC -3′; R, 5′- TCCACACGTCCAGAACAGTC -3′; HPRT: F, 5′- GACCGGTCCCGTCATGC -3′; R, 5′- TCATAACCTGGTTCATCATCGC -3′. F, forward primer; R, reverse primer. Flow cytometry Cells were stained with Abs specific for mouse TCRβ, F4/80, CD11b, CD11c, CD40, CD64, CD80, CD86, Ly6G, Siglec-F, CD4, Foxp3, IL-17, IFN-γ, pro-IL-1β or with isotype-matched controls (1:100 dilution for each antibody; BD Pharmingen or eBiosciences) and analysed using a FACSCalibur or LSRII flow cytometer with Cell Quest (BD Biosciences) or FlowJo (TreeStar) softwares. BRDU staining Mice were injected i.p. with 150 μl BrdU (10 mg ml −1 ) in sterile 1 × DPBS. After 16–20 h, lymphocytes were isolated, stained with Abs to cell surface markers, fixed and permeabilized with Cytofix/Cytoperm Buffer (BD Biosciences), treated with DNase (300 μg ml −1 ) at 37 °C for 1 h, stained with anti-BrdU-APC (BD BRDU flow kit) and analysed by flow cytometry. BMDM culture and LPS stimulation BMDMs were generated by culturing mouse bone marrow cells in L-cell-conditioned IMDM. The L-cell-conditioned medium comprised supernant from cultures of L929 cells secreting M-CSF mixed at a 1:2 ratio with IMDM and then supplemented with 10% FBS, 1% nonessential amino acids and 1% penicillin–streptomycin. After 6 days of culture, cells were seeded in 12-well plates, and the next day treated with IL-10 (50 ng ml −1 ) or anti-IL-10Rα Ab (1 μg ml −1 ), and 4 h later stimulated with or without LPS (20 ng ml −1 ) for 12 h. For the final 30 min, 5 mM ATP was added into the medium [53] . Western blot Culture samples were denatured in loading buffer containing SDS and 100 mM dithiothreitol, and boiled for 5 min. SDS–PAGE-separated proteins were transferred to polyvinylidene difluoride membranes and immunoblotted with primary Abs against caspase-1 (Adipogen; AG-20B-0042 or kind gift of Dr Peter Vandenabeele, Ghent University), IL-1β (R&D Systems) and GAPDH (Cell Signaling Technology; D16H11), followed by secondary anti-rabbit, anti-rat, anti-mouse or anti-goat horse radish peroxidase (HRP) Abs (Jackson ImmunoResearch Laboratories) [54] . Images have been cropped for presentation. Full-size images are presented in Supplementary Fig. 7 . Th17 culture Naive (CD4 + CD45RB high CD25 − ) T cells were purified by cell sorting to a purity >99%. These (5 × 10 5 ) were co-cultured at a ratio of 5:1 with or without sorted LPMφs from 8-week-diseased IL-10Rα Mdel Rag1 −/− or Rag1 −/− mice in 96-well plates pre-coated with 1 μg ml −1 anti-CD3 and 2 μg ml −1 anti-CD28. Cells were cultured in complete RPMI 1640 media containing 5 ng ml −1 TGF-β, 10 μg ml −1 anti-IL-4 and 10 μg ml −1 anti-IFN-γ Abs. In all, 20 ng ml −1 IL-6 was added to a positive control Th17 culture condition only. After 4 days, cells were washed and restimulated with cytokine stimulation cocktail containing phorbol myristate acetate, Ionomycin and Brefeldin A (Cell stimulation cocktail, eBioscience) for 4 h at 37 °C. Cells were washed and stained for the indicated cytokines. Immunohistochemistry Tissue cryosections were fixed in 4% paraformaldehyde (PFA) at 4 °C overnight, embedded in optimal cutting temperature compound and sectioned in a cryostat (12 μm). For IL-1β immunostaining, sections were incubated with a polyclonal goat anti-mouse IL-1β primary antibody (1:200, R&D Systems) and monoclonal rat anti-mouse CD11b antibody (1:500, AbD Serotec). After washing three times with TBST, sections were incubated with Cy3-labelled donkey-anti-rat IgG antibody (1:200, Jackson Lab) and Alexa 488-labelled donkey anti-goat IgG antibody (1:200, Molecular Probes). Sections were mounted with mounting medium containing DAPI (Invitrogen) and confocal microscopy was performed. Statistics Statistics were calculated using Prism5 (GraphPad Software). Group comparisons were by two-sided Student’s t -test or, when multiple cohorts were present, analysis of variance with Bonferroni correction. A P <0.05 was considered significant. How to cite this article: Li, B. et al . IL-10 engages macrophages to shift Th17 cytokine dependency and pathogenicity during T-cell-mediated colitis. Nat. Commun. 6:6131 doi: 10.1038/ncomms7131 (2015).